Multi-protein assemblies underlie the mesoscale organization of the plasma membrane Most proteins have uneven distributions in the plasma membrane. Broadly speaking, this may be caused by mechanisms specific to each protein, or may be a consequence of a general pattern that affects the distribution of all membrane proteins. The latter hypothesis has been difficult to test in the past. Here, we introduce several approaches based on click chemistry, through which we study the distribution of membrane proteins in living cells, as well as in membrane sheets. We found that the plasma membrane proteins form multi-protein assemblies that are long lived (minutes), and in which protein diffusion is restricted. The formation of the assemblies is dependent on cholesterol. They are separated and anchored by the actin cytoskeleton. Specific proteins are preferentially located in different regions of the assemblies, from their cores to their edges. We conclude that the assemblies constitute a basic mesoscale feature of the membrane, which affects the patterning of most membrane proteins, and possibly also their activity. The introduction of far-field super-resolution light microscopy has revealed the nanoscale organization of an impressive array of proteins in mammalian cells, ranging from plasma membrane proteins to nuclear ones [1] , [2] , [3] , [4] . Interestingly, most of the proteins observed in the plasma membrane form nanoscale domains or clusters, typically of the order of a few tens of nanometres, whose assembly is thought to depend on the characteristics of each protein. While the nanoscale organization of specific proteins has been determined in great detail, a putative mesoscale organization of the proteins, and its connection to the nanoscale domains, has been studied less intensively. At first glance, the domains of abundant proteins may appear to be distributed randomly across the membrane, for example, for syntaxin 1 (ref. 5 ), syntaxin 4 (ref. 6 ), SNAP25 (refs 7 , 8 ), synaptotagmin 1 (ref. 9 ), synaptophysin [10] , synaptobrevin 2 (ref. 5 ) or amyloid precursor protein [11] . However, when inspecting the protein distributions more carefully, a non-random mesoscale pattern becomes apparent [1] , [5] , [7] , [8] , [9] , [11] , [12] . The protein domains do not spread evenly on the entire membrane, but gather in small, irregularly shaped areas with a breadth of up to a few hundred nanometres. These are separated from other such areas by narrow regions in which proteins are virtually absent. The observation of such patterns for several types of proteins suggests that a common mechanism affects them all. The simplest explanation for the observed patterns is the formation of protein-enriched areas in the plasma membrane. Indeed, this has been hypothesized in the past, based on the observation of a patchwork of electron-dense and light areas in osmium-stained isolated plasma membranes (for example, refs 13 , 14 , 15 , 16 ). The dense areas were shown to co-localize with different types of proteins, leading to the suggestion that they represent ‘protein islands’ that contain most of the membrane proteins [15] (although osmium staining may not reveal just the protein distribution [17] ). Yet, it is still difficult to estimate whether membrane proteins are patterned into general protein-rich domains in living cells, or whether this is only a membrane isolation artefact. Although this type of membrane arrangement has been supported by several live-cell single-molecule imaging studies [12] , [18] , and different general mechanisms based on the membrane skeleton and membrane rafts have been suggested [19] , [20] , [21] , a systematic characterization of the mesoscale protein organization and its relation to nanoscale protein domains in mammalian cell membranes is still missing. Here, we analysed the distribution of proteins by several approaches based on metabolic labelling and click chemistry, both in living cells and in membrane sheets. We found that plasma membrane proteins were not homogeneously distributed in living cells. They formed assemblies where protein diffusion was constrained, and which persisted on a time scale of at least several minutes. Isolation of membrane sheets allowed a more thorough investigation of these assemblies, without seeming to change their organization in a fundamental fashion. We found that the protein assemblies were stabilized by cholesterol and, to a lesser extent, by actin. Specific proteins preferred different positions in these assemblies, often overlapping with several of their functional partners. This suggests that the assemblies are a basic mesoscale form of membrane patterning, on which more specific interactions may build functional domains. Plasma membranes of living cells feature protein assemblies To visualize the general organization of membrane proteins, it is necessary to label a representative fraction of all proteins indiscriminately, and to detect them with sufficient sensitivity and resolution. We relied on the metabolic incorporation of a modified amino acid, L-Azidohomoalanine (AHA), which replaces endogenous methionine in newly produced proteins [22] . Monkey kidney fibroblast cells (COS-7) or rat neuroendocrine cells (PC12) were grown for several days with AHA, allowing its incorporation into a substantial fraction of cellular proteins, without negative effects on membrane trafficking, cellular morphology and organelle and protein distribution. To investigate the distribution of plasma membrane proteins in living cells, AHA moieties incorporated into proteins exposed on the outer surface of the cells were coupled to the fluorophore KK114 conjugated to aza-dibenzocyclooctyne (DIBAC [23] ), using a copper-free strain-promoted azide-alkyne cycloaddition (click reaction) [24] , [25] performed for 1 h under physiological conditions ( Fig. 1a ). We imaged the cells using two-colour stimulated emission depletion (STED) microscopy [9] , [26] at 37 °C. STED microscopy was preferred to stochastic approaches such as PALM, STORM or GSDIM [3] , since STED does not rely on computational post-processing for image reconstruction [27] , [28] ). We detected a patterned protein distribution ( Fig. 1b,c ), which correlated poorly with the overall distribution of a membrane lipid probe ( Fig. 1c ). This suggests that the pattern represents the localization of proteins, rather than membrane-attached vesicular material or membraneous formations (infoldings, ruffles). 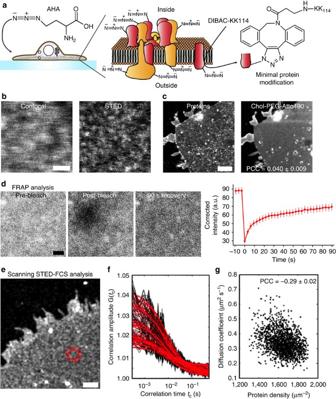Figure 1: Proteins are organized into assemblies in the plasma membrane of living cells. (a) The general principle of the protein labelling. The amino acid L-AHA is metabolically incorporated into cells for 72 h. The fluorophore DIBAC-KK114 is then covalently coupled to the proteins on the outer surface of COS-7 cells through a copper-free click reaction, allowing live investigation by various imaging approaches at 37 °C. (b) Confocal and STED micrographs of the protein organization in the membrane of living cells. Note the areas with high abundance of proteins (protein assemblies). Scale bar, 500 nm. (c) STED micrographs of plasma membrane proteins (DIBAC-KK114) and a lipid probe, cholesterol-polyethyleneglycol(PEG)-Atto490LS. The lipid probe is homogeneously distributed, few exceptions likely representing organelles or membrane infoldings. The correlation of the protein and lipid labelling is low; the Pearson correlation coefficient (PCC) is 0.040±0.009 (mean±s.e.m.,n=9 cells). Scale bar, 2 μm. (d) Analysis of protein mobility by FRAP. A confocal image sequence displays the protein signal before (‘pre-bleach’) and immediately after (‘post-bleach’) photobleaching, and after 90 s of recovery. Scale bar, 1 μm. The change of intensity over time is plotted after background subtraction and correction for imaging-induced bleaching (mean±s.e.m.,n=87 recovery traces from 30 cells in three independent experiments). (e) Analysis of protein mobility by scanning STED-FCS measurements. The confocal micrograph shows the overview of the bottom membrane of a living COS-7 cell. Scale bar, 2 μm. The detection spot (90 nm in diameter) was continuously scanned (4 kHz) on a circular trajectory (red circle) over the membrane. (f) The scanning trajectory was subdivided into 50 pixels, and a temporal autocorrelation analysis was performed on each pixel. The correlation curves were fitted (red) according to the standard two-dimensional FCS diffusion model. From the fit for each position along the scanning trajectory, the amplitude and the half-time of decay were obtained, which were used to calculate the local protein density and diffusion coefficient, respectively. (g) Scatter plot of the protein density against the protein mobility (diffusion coefficientD) shows a significant negative correlation. The PCC is −0.29±0.02 (mean±s.d.,n=500 data points from 10 cells in three independent preparations). Figure 1: Proteins are organized into assemblies in the plasma membrane of living cells. ( a ) The general principle of the protein labelling. The amino acid L-AHA is metabolically incorporated into cells for 72 h. The fluorophore DIBAC-KK114 is then covalently coupled to the proteins on the outer surface of COS-7 cells through a copper-free click reaction, allowing live investigation by various imaging approaches at 37 °C. ( b ) Confocal and STED micrographs of the protein organization in the membrane of living cells. Note the areas with high abundance of proteins (protein assemblies). Scale bar, 500 nm. ( c ) STED micrographs of plasma membrane proteins (DIBAC-KK114) and a lipid probe, cholesterol-polyethyleneglycol(PEG)-Atto490LS. The lipid probe is homogeneously distributed, few exceptions likely representing organelles or membrane infoldings. The correlation of the protein and lipid labelling is low; the Pearson correlation coefficient (PCC) is 0.040±0.009 (mean±s.e.m., n =9 cells). Scale bar, 2 μm. ( d ) Analysis of protein mobility by FRAP. A confocal image sequence displays the protein signal before (‘pre-bleach’) and immediately after (‘post-bleach’) photobleaching, and after 90 s of recovery. Scale bar, 1 μm. The change of intensity over time is plotted after background subtraction and correction for imaging-induced bleaching (mean±s.e.m., n =87 recovery traces from 30 cells in three independent experiments). ( e ) Analysis of protein mobility by scanning STED-FCS measurements. The confocal micrograph shows the overview of the bottom membrane of a living COS-7 cell. Scale bar, 2 μm. The detection spot (90 nm in diameter) was continuously scanned (4 kHz) on a circular trajectory (red circle) over the membrane. ( f ) The scanning trajectory was subdivided into 50 pixels, and a temporal autocorrelation analysis was performed on each pixel. The correlation curves were fitted (red) according to the standard two-dimensional FCS diffusion model. From the fit for each position along the scanning trajectory, the amplitude and the half-time of decay were obtained, which were used to calculate the local protein density and diffusion coefficient, respectively. ( g ) Scatter plot of the protein density against the protein mobility (diffusion coefficient D ) shows a significant negative correlation. The PCC is −0.29±0.02 (mean±s.d., n =500 data points from 10 cells in three independent preparations). Full size image Fluorescence recovery after photobleaching (FRAP) experiments, performed with conventional confocal microscopy, demonstrated that molecules forming the pattern were relatively dynamic ( Fig. 1d ). We observed a 67%±3% recovery within ~90 s (mean±s.e.m., n =87 recovery traces from 30 cells, three independent experiments), composed of an initial rapid phase (with a half-time of 3.6 s, from a double exponential fit of the recovery curve), which accounted for about half of the recovery, and of a slow, almost linear phase (with a longer half-time of 64.2 s). The diffusion coefficients for these two protein populations were 0.22 and 0.01 μm 2 s −1 , respectively. As confocal FRAP experiments lacked the spatiotemporal resolution required to observe diffusion heterogeneities in detail, we turned to fluorescence correlation spectroscopy in combination with STED (STED-FCS). In these experiments, we constantly scanned the detection spot on a circular trajectory [29] over the plasma membrane at high frequency (4 kHz; Fig. 1e ). This scanning modality allowed us to determine both the local mobility and the density of proteins along multiple positions on the membrane, simultaneously, with a spatial resolution of 100 nm. As in conventional FCS, the average number and the mobility of the fluorescent proteins was determined by correlation analysis of the intensity fluctuations stemming from the diffusion of labelled proteins through the observation spot [30] . But instead of a single correlation curve per measurement, we obtained 50 curves per scanning STED-FCS measurement, representing spatially separated (100 nm) positions on the scan trajectory ( Fig. 1f ). The correlation analysis can be accurately applied up to a density of 50 fluorescent molecules per observation spot. Unfortunately, as for any FCS measurement, slowly moving or immobilized particles cannot be detected, since they do not cross the observation spot and therefore cause no intensity fluctuations. We found that the local diffusion coefficient ( D ) and the density of labelled proteins ( c ) varied with D =0.1–0.6 μm 2 s −1 and c =1,000–2,000 proteins per μm 2 over the positions on the scanning trajectories. To analyse the dependence of D on the protein density, we plotted a two-dimenisonal scatter graph, and calculated the Pearson correlation coefficient ( Fig. 1g ). We found a significant negative correlation, which indicates that diffusion was restricted at high protein density sites. Taking into account that the scanning STED-FCS experiments were only sensitive to the highly mobile fraction of molecules, the observed relation between local protein density and protein mobility is probably an underestimation. Our scanning STED-FCS results are in line with previous observations for proteins in the outer membrane leaflet [31] . Altogether, our mobility measurements indicate that areas of high protein density are correlated with low protein diffusion. Cell–cell fusion confirms the presence of stable assemblies We next sought to verify the presence of such protein assemblies and designed a multicolour labelling experiment that examines the intermixing of proteins. One set of cells was grown in presence of AHA, while a second set received another methionine analogue, homopropargylglycine (HPG; Fig. 2a ). We then induced the cells to fuse using inactivated Sendai virus particles [32] , and allowed fusion to proceed for 5–10 min. To investigate the plasma membrane in the absence of adjacent cytoplasmic structures, and to allow the labelling of proteins on both sides of the membrane, after cell fusion, we applied a sonication procedure that isolates the substrate-attached plasma membrane sheets [33] ( Fig. 2a ). The membranes were chemically fixed, and the two amino acid analogues were coupled to two different fluorescent dyes through sequential click reactions, followed by imaging with two-colour STED microscopy. 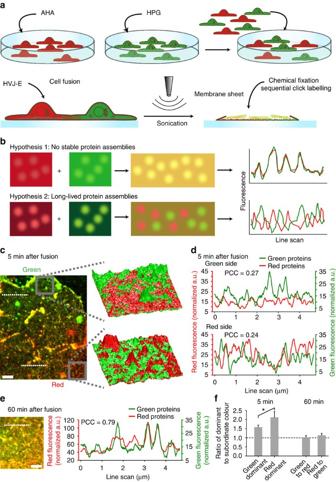Figure 2: Cell–cell fusion experiments show that protein assemblies are long-lived. (a) COS-7 cells that incorporated methionine analogues, AHA (red) or HPG (green) for 60 h were plated together and cell–cell fusion was induced by HVJ-E. Membrane sheets were generated from the fused cells, fixed, and labelled by click reaction. (b) Two possible scenarios are anticipated. Top, in absence of stable assemblies, the fused membrane would contain both red and green proteins with similar distributions. A line scan through the membrane would show that the green and red signals correlate. Bottom, if long-lived assemblies exist, then the fused membrane would initially contain red assemblies that exclude green proteins, and vice versa. The areas between the assemblies should contain more mobile proteins that intermix faster. (c) Two-colour STED image of a typical membrane sheet obtained after fusion. Following fusion, cells were incubated at 37 °C for 5 min before generation and fixation of membrane sheets. The three-dimensional views (prepared using a metallic, non-transparent colourmap in Matlab) show the signal distributions for an HPG-dominated area (top) and AHA-dominated area (bottom). (d) 4.65 μm long (three-pixels wide) line scans were drawn through green (top) or red (bottom) protein assemblies, at the positions indicated by the dashed lines inc. Note the low correlation of red proteins with green assemblies, and similarly of green proteins with red assemblies. (e) Alternatively, following fusion, cells were further incubated for 60 min. Line scans were drawn as ind, at the position marked by the dashed line. Note the increased correlation. Scale bars, 2 μm. (f) Using line scans, we analysed the enrichment of red- and green-labelled proteins in the assemblies of the opposite colour (normalized to their own baseline). At 5 min, the dominant protein is substantially more enriched in its own assemblies than the subordinate colour (for the green side of the fused membrane, green is dominant and red is subordinate). The differences were statistically significant (*P<0.05,t-tests). At 60 min, there is no clear dominance, so the same regions of interest were analysed either with normalization to green or red signal. The enrichment was much more even (n=15–19 fused cells from three independent experiments). Figure 2: Cell–cell fusion experiments show that protein assemblies are long-lived. ( a ) COS-7 cells that incorporated methionine analogues, AHA (red) or HPG (green) for 60 h were plated together and cell–cell fusion was induced by HVJ-E. Membrane sheets were generated from the fused cells, fixed, and labelled by click reaction. ( b ) Two possible scenarios are anticipated. Top, in absence of stable assemblies, the fused membrane would contain both red and green proteins with similar distributions. A line scan through the membrane would show that the green and red signals correlate. Bottom, if long-lived assemblies exist, then the fused membrane would initially contain red assemblies that exclude green proteins, and vice versa. The areas between the assemblies should contain more mobile proteins that intermix faster. ( c ) Two-colour STED image of a typical membrane sheet obtained after fusion. Following fusion, cells were incubated at 37 °C for 5 min before generation and fixation of membrane sheets. The three-dimensional views (prepared using a metallic, non-transparent colourmap in Matlab) show the signal distributions for an HPG-dominated area (top) and AHA-dominated area (bottom). ( d ) 4.65 μm long (three-pixels wide) line scans were drawn through green (top) or red (bottom) protein assemblies, at the positions indicated by the dashed lines in c . Note the low correlation of red proteins with green assemblies, and similarly of green proteins with red assemblies. ( e ) Alternatively, following fusion, cells were further incubated for 60 min. Line scans were drawn as in d , at the position marked by the dashed line. Note the increased correlation. Scale bars, 2 μm. ( f ) Using line scans, we analysed the enrichment of red- and green-labelled proteins in the assemblies of the opposite colour (normalized to their own baseline). At 5 min, the dominant protein is substantially more enriched in its own assemblies than the subordinate colour (for the green side of the fused membrane, green is dominant and red is subordinate). The differences were statistically significant (* P <0.05, t -tests). At 60 min, there is no clear dominance, so the same regions of interest were analysed either with normalization to green or red signal. The enrichment was much more even ( n =15–19 fused cells from three independent experiments). Full size image Two scenarios could, in principle, be envisaged for this experiment. In the first case ( Fig. 2b , top panels), the proteins in the plasma membrane do not form stable assemblies. Fusion of the membranes would lead to intermixing of AHA- and HPG-labelled proteins, resulting in a similar pattern of distribution. This would be the case even if the generation of plasma membrane sheets induces artificial protein clustering, since these would form only after protein intermixing, and would thus be similarly labelled by both amino acids. In the second case ( Fig. 2b , bottom panels), the plasma membrane contains protein assemblies that are long-lived (at least a few minutes), and thus cannot exchange rapidly with neighbouring proteins. This situation would lead to the exclusion of proteins with one type of label from the assemblies of the opposite label. The space between the protein assemblies, which is occupied by more mobile proteins (as suggested by Fig. 1 ), would contain both labels. Our experimental data supported only the second scenario ( Fig. 2c ). The membrane sheets from fused cells typically contained a side dominated by AHA (red in Fig. 2c ), which was presumably derived from an AHA-labelled cell, and one dominated by HPG (green in Fig. 2c ). The AHA-dominated part of the membrane contained numerous AHA-labelled protein assemblies, surrounded by a more protein-poor space that was occupied by both AHA- and HPG-labelled proteins ( Fig. 2c,d ). The opposite was observed in the HPG-dominated part of the membrane. To test whether the two sets of proteins eventually intermix, cells were incubated for longer time after fusion (up to 60 min). The longer incubation indeed resulted in a much higher correlation and more even intermixing for the two sets of proteins ( Fig. 2e ). On average, for the 5-min time point the assemblies were 1.5- to twofold more enriched for the dominant colour (meaning, AHA in the AHA-dominated side of the membrane) than for the subordinate one, confirming that the intermixing of proteins from the assemblies is slow ( Fig. 2f ). An almost fully intermixed state can be observed at 60 min after fusion ( Fig. 2e,f ). This observation confirms the suggestions from our protein mobility analyses ( Fig. 1d–g ), namely that plasma membrane protein assemblies do exist in living cells. Moreover, they are relatively long-lived, since they persist for at least several minutes after membrane fusion. Protein assemblies concentrate different classes of proteins As shown in Fig. 2 , membrane sheets can be used to visualize protein assemblies, which makes them an attractive model system. Protein assemblies had a more pronounced appearance in fixed plasma membrane sheets, in comparison with the living cells ( Fig. 3a ). The size of the assemblies also appeared larger than in living cells ( Fig. 3b ). This may partially be due to the fact that the contrast of the images is higher in membrane sheets, as a result of more efficient copper-catalysed click reaction operating on both sides of the membrane (which cannot be applied to intact living cells). In addition, the image contrast in live cells at 37 °C is limited by the rapid diffusion of molecules. Similar results were observed for unfixed sheets, or under different fixation schemes (either with paraformaldehyde (PFA) alone or in combination with glutaraldehyde, applied before or after the generation of the sheets; Supplementary Fig. 1a–c ). 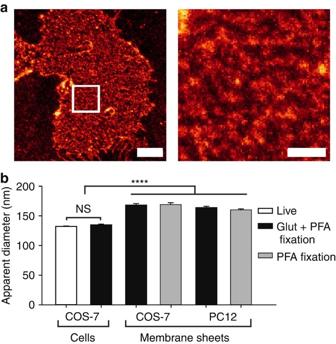Figure 3: Protein assemblies in plasma membrane sheets. (a) Left, STED micrograph of the protein organization in PC12 membrane sheets. AHA was metabolically incorporated into PC12 cells for 72 h before generation of membrane sheets. The sheets were then fixed and subject to copper-catalysed click reaction with alkyne-functionalized Atto647N. Right, a high-zoom view of the area marked with the white square on the left. Scale bars, 2 μm and 500 nm. SeeSupplementary Fig. 1a–cfor controls showing the protein labelling specificity, and the reproducibility of the protein pattern under different fixation schemes. (b) The graph shows the assembly size (apparent diameter) for protein assemblies from live and fixed cells, and from membrane sheets (NS, non-significant; ****P<0.0001, 1-way analysis of variance, Bonferroni’s multiple comparison test,n=573–6,812 protein assemblies. SeeSupplementary Methodsfor details of the analysis. Figure 3: Protein assemblies in plasma membrane sheets. ( a ) Left, STED micrograph of the protein organization in PC12 membrane sheets. AHA was metabolically incorporated into PC12 cells for 72 h before generation of membrane sheets. The sheets were then fixed and subject to copper-catalysed click reaction with alkyne-functionalized Atto647N. Right, a high-zoom view of the area marked with the white square on the left. Scale bars, 2 μm and 500 nm. See Supplementary Fig. 1a–c for controls showing the protein labelling specificity, and the reproducibility of the protein pattern under different fixation schemes. ( b ) The graph shows the assembly size (apparent diameter) for protein assemblies from live and fixed cells, and from membrane sheets (NS, non-significant; **** P <0.0001, 1-way analysis of variance, Bonferroni’s multiple comparison test, n =573–6,812 protein assemblies. See Supplementary Methods for details of the analysis. Full size image As membrane sheets also allow the efficient control of experimental conditions, we continued to use them to investigate the organization principles of the protein assemblies. We restricted our analysis to flat membrane areas, free of attached organelles, as demonstrated by lipid staining of the membranes (using the lipid tracer octadecyl rhodamine B). We first tested whether proteins of different ages accumulate to the same assemblies, by incubating the cells first with AHA, for 72 h, to label most of the cellular proteins, and then with HPG, for 3 h, to label only the most recently synthesized proteins. Both amino acids localized to the same assemblies ( Fig. 4a ), although the new, recently synthesized proteins (revealed by HPG) did not enrich to the same extent in the centres. The same was observed when we reversed the fluorophores for AHA and HPG coupling ( Fig. 4a ). This result could be related to the lower penetration of new proteins into the more crowded centres of protein assemblies, which feature slow exchange rates (as already suggested by Figs 1g and 2 ). 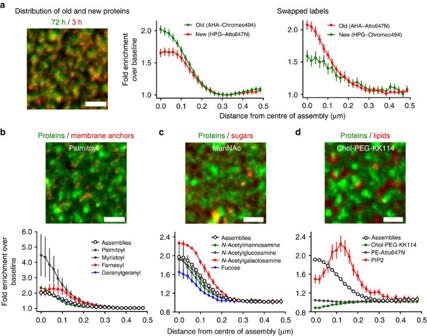Figure 4: Protein assemblies in membrane sheets contain proteins of different ages and classes. (a) Two-colour STED imaging of proteins of different ages. PC12 cells were incubated first with AHA for 72 h (old proteins, green), then starved of methionine for 1 h, and incubated with HPG for 3 h (new proteins, red). Two click reactions were applied sequentially coupling first HPG to Atto647N-azide, then AHA to Chromeo494-alkyne. To analyse the relative distributions of the two labels line scans centred on the green AHA spots were performed. After normalization to the baseline, the scans were aligned using their maxima in the green channel as reference. The graph on the left shows averaged line scans from 856 protein assemblies (mean±s.e.m.). Note that the newer proteins are less strongly enriched in the centres of assemblies. The same observation was made when the two fluorophores are swapped (graph on the right), coupling AHA to Atto647N-alkyne (old, red) and HPG to Chromeo494-azide (new, green),n=768 assemblies. (b,c) Distributions of different classes of post-translationally modified proteins (red) carrying various membrane anchors (b) or glycosylations (c), with respect to general protein assemblies (green). In addition to AHA or HPG, PC12 cells were treated with clickable versions of the indicated post-translational modifiers, and were sequentially labelled by click reactions. A typical two-colour STED image for palmitoyl labelling is shown. For each condition, a plot was generated as described above.n=3–4 independent experiments, with a total of 629–1,373 analysed protein assemblies. A reference trace for the protein assemblies (black hollow circles) was obtained by averaging the protein profiles from all the conditions represented in each graph. SeeSupplementary Fig. 2for the analysis of the GPI-anchor. (d) Distribution of lipid probes in relation to protein assemblies. After click labelling of proteins with Chromeo494, membrane sheets were incubated with cholesterol-PEG-KK114 or Atto647N-PE at RT for 30 min (seeSupplementary Methodsfor more information about the lipid probes). A typical image for cholesterol analogue is shown. Alternatively, phophatidyl-inositol 4,5-bisphosphate (PIP2) was probed through immunostaining (seeSupplementary Methods). For the two fluorescent lipid analogues,n=3–4 independent experiments, with a total of 1,373–1,675 protein assemblies. For PIP2 immunostaining,n=285 assemblies. The error bars are occasionally smaller than the data point symbols. Scale bar, 750 nm. Figure 4: Protein assemblies in membrane sheets contain proteins of different ages and classes. ( a ) Two-colour STED imaging of proteins of different ages. PC12 cells were incubated first with AHA for 72 h (old proteins, green), then starved of methionine for 1 h, and incubated with HPG for 3 h (new proteins, red). Two click reactions were applied sequentially coupling first HPG to Atto647N-azide, then AHA to Chromeo494-alkyne. To analyse the relative distributions of the two labels line scans centred on the green AHA spots were performed. After normalization to the baseline, the scans were aligned using their maxima in the green channel as reference. The graph on the left shows averaged line scans from 856 protein assemblies (mean±s.e.m.). Note that the newer proteins are less strongly enriched in the centres of assemblies. The same observation was made when the two fluorophores are swapped (graph on the right), coupling AHA to Atto647N-alkyne (old, red) and HPG to Chromeo494-azide (new, green), n =768 assemblies. ( b , c ) Distributions of different classes of post-translationally modified proteins (red) carrying various membrane anchors ( b ) or glycosylations ( c ), with respect to general protein assemblies (green). In addition to AHA or HPG, PC12 cells were treated with clickable versions of the indicated post-translational modifiers, and were sequentially labelled by click reactions. A typical two-colour STED image for palmitoyl labelling is shown. For each condition, a plot was generated as described above. n =3–4 independent experiments, with a total of 629–1,373 analysed protein assemblies. A reference trace for the protein assemblies (black hollow circles) was obtained by averaging the protein profiles from all the conditions represented in each graph. See Supplementary Fig. 2 for the analysis of the GPI-anchor. ( d ) Distribution of lipid probes in relation to protein assemblies. After click labelling of proteins with Chromeo494, membrane sheets were incubated with cholesterol-PEG-KK114 or Atto647N-PE at RT for 30 min (see Supplementary Methods for more information about the lipid probes). A typical image for cholesterol analogue is shown. Alternatively, phophatidyl-inositol 4,5-bisphosphate (PIP2) was probed through immunostaining (see Supplementary Methods ). For the two fluorescent lipid analogues, n =3–4 independent experiments, with a total of 1,373–1,675 protein assemblies. For PIP2 immunostaining, n =285 assemblies. The error bars are occasionally smaller than the data point symbols. Scale bar, 750 nm. Full size image We followed a similar click-based procedure to test the localization of proteins with different post-translational modifications with respect to the general protein assemblies. Using commercially available clickable modifiers, we assayed subsets of modified proteins with different lipid anchors (palmitoyl, farnesyl, myristoyl, geranylgeranyl), and glycosylations ( N -acetylglucosamine, N -acetylgalactosamine, N -acetylmannosamine, fucose), by two-colour STED microscopy (see Methods). We also investigated the distribution of a model glycophosphatidylinositol (GPI)-anchored protein ( Supplementary Fig. 2 ), by expressing the acyl carrier protein (ACP) with a GPI anchor signal sequence, and fluorescently labelling it via the ACP-synthase reaction. As indicated in Fig. 4b,c and Supplementary Fig. 2 , all of the differently modified protein populations co-localized to the general protein assemblies. The degrees of enrichment ranged from 1.2 for GPI–ACP to 4.5 for myristoylated proteins. Occasionally, distributions showed variations from those of general proteins. For example, the palmitoylated proteins were located especially in the centres, forming a tighter distribution than general proteins (lateral spread 30% smaller; four independent experiments), while farnesylated proteins showed a slightly broader distribution ( Fig. 4b ). All glycosylated proteins followed the pattern of the general protein distribution ( Fig. 4c ). Unlike the proteins, fluorophore-coupled analogues of lipids showed a much more homogeneous and random distribution in membrane sheets of PC12 cells ( Fig. 4d ). An Atto647N-coupled phosphatidylethanolamine (PE) analogue did not show any enrichment in the assemblies, whereas a KK114-coupled cholesterol analogue slightly avoided the assembly centres ( Fig. 4d ). Phophatidyl-inositol 4,5-bisphosphate (PIP2), a more specialized lipid that is known to interact with several proteins, was found by immunostaining mostly at the edges of the protein assemblies ( Fig. 4d ), possibly as a result of interactions with specific proteins (see below). Overall, localization in the protein assemblies does not seem to be a feature of proteins with a particular modification or membrane anchor. On the contrary, a variety of proteins seem to be enriched in the assemblies (albeit at different levels). Lipids in general are not enriched in the assemblies, confirming that the higher intensity of protein labelling is not merely due to higher amounts of membrane material in these areas (as also expected from the lipid staining shown in Fig. 1c ). The protein pattern in membranes resists most perturbations The observations presented above suggest that protein assemblies are relatively long-lived and contain various types of proteins. To test their stability, we subjected membrane sheets to many harsh treatments proposed to influence the patterning of many subgroups of membrane proteins: strong increases or decreases in ionic strength, abrupt changes in Ca 2+ concentration, hydrolysis of sphingomyelin by applying the enzyme sphingomyelinase (SPMase) or hydrolysis of other lipids by phospholipases A2, C and D ( Fig. 5a,b ). Furthermore, several treatments were applied onto full cells before sonication, including intracellular modulation of Ca 2+ concentration by ionomycin, reduction of protein crowding by knocking down abundant membrane proteins (syntaxin 1 and SNAP25) or microtubule dispersion ( Fig. 5c ). To perturb the actin cytoskeleton, cells were treated with actin-depolymerizing drugs such as latrunculin A or cytochalasin D ( Fig. 5c ). In comparison with the control conditions, neither of these treatments had a significant effect on the overall area occupied by the protein assemblies (see analysis in Supplementary Methods ; Fig. 5d ), indicating that they could not alter the forces grouping proteins within the assemblies. Finally, the overexpression of syntaxin 1 and SNAP25 did not affect the overall membrane pattern, although a small (but significant) increase was observed in the relative intensity of the areas with low protein abundance ( Supplementary Fig. 3a–c ). 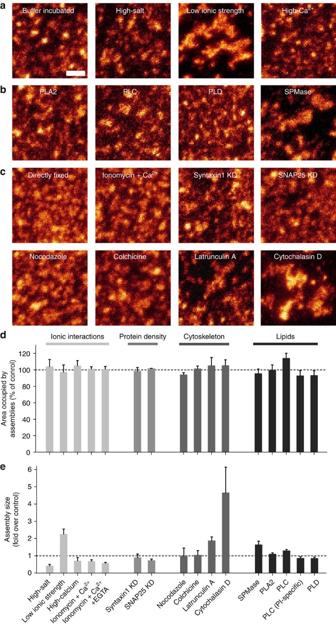Figure 5: Protein assembly organization persists after many harsh treatments. STED images of protein assemblies in PC12 membrane sheets subjected to different treatments either applied on sheets before fixation (a,b) or onto live cells before generation of sheets (c). (a) Membrane sheets were either incubated in sonication buffer (which mimics the intracellular conditions, leftmost image) as control or treated with buffers of high-salt, low ionic strength or high-calcium, for 20 min at 37 °C (see Methods for buffer compositions). Scale bar, 500 nm. (b) Lipid composition of the membranes was manipulated by applying 1–2 units ml−1phospholipases (PL) A2, C, D and phosphatidylinositol (PI)-specific PLC (not shown) or 20 units ml−1SPMase diluted in sonication buffer, for 15 min. Compare with the first image ina(albeit incubated for 20 min, rather than 15 min; an image of a 15-min incubated membrane sheet is shown inFig. 6a). (c) For treatments on full cells, controls were prepared by chemically fixing the membrane sheets directly after sonication. For ionic perturbation, cells were treated for 5 min with 1 μM of ionomycin in HEPES-buffered medium containing 5 mM Ca2+, with or without 10 mM EGTA. In independent experiments, the abundant membrane proteins syntaxin 1 or SNAP25 were knocked down by siRNAs. See alsoSupplementary Fig. 3a–cfor the effect of overexpression of proteins. To manipulate the cytoskeletal elements, cells were treated for 1 h with 0.1% dimethyl sulfoxide (as solvent control, not shown), 10 μM nocodazole, colchicine or cytochalasin D or 1 μM latrunculin A. (d) For all the conditions, the area occupied by assemblies was quantified and expressed as % of the respective control for each condition. (e) The graph indicates the assembly sizes (average assembly area) for each condition as fold increase over their respective control conditions. (d,e)n=3–5 independent experiments, means±s.e.m. for all treatments, except for the knockdown (KD) conditions, where means±range of values (from two independent experiments) are shown. Data analyses are explained in theSupplementary Methods. The strongest increases in size are seen under treatments of low ionic strength, SPMAse, latrunculin A or cytochalasin D, all of which affect the membrane actin cytoskeleton. Figure 5: Protein assembly organization persists after many harsh treatments. STED images of protein assemblies in PC12 membrane sheets subjected to different treatments either applied on sheets before fixation ( a , b ) or onto live cells before generation of sheets ( c ). ( a ) Membrane sheets were either incubated in sonication buffer (which mimics the intracellular conditions, leftmost image) as control or treated with buffers of high-salt, low ionic strength or high-calcium, for 20 min at 37 °C (see Methods for buffer compositions). Scale bar, 500 nm. ( b ) Lipid composition of the membranes was manipulated by applying 1–2 units ml −1 phospholipases (PL) A2, C, D and phosphatidylinositol (PI)-specific PLC (not shown) or 20 units ml −1 SPMase diluted in sonication buffer, for 15 min. Compare with the first image in a (albeit incubated for 20 min, rather than 15 min; an image of a 15-min incubated membrane sheet is shown in Fig. 6a ). ( c ) For treatments on full cells, controls were prepared by chemically fixing the membrane sheets directly after sonication. For ionic perturbation, cells were treated for 5 min with 1 μM of ionomycin in HEPES-buffered medium containing 5 mM Ca 2+ , with or without 10 mM EGTA. In independent experiments, the abundant membrane proteins syntaxin 1 or SNAP25 were knocked down by siRNAs. See also Supplementary Fig. 3a–c for the effect of overexpression of proteins. To manipulate the cytoskeletal elements, cells were treated for 1 h with 0.1% dimethyl sulfoxide (as solvent control, not shown), 10 μM nocodazole, colchicine or cytochalasin D or 1 μM latrunculin A. ( d ) For all the conditions, the area occupied by assemblies was quantified and expressed as % of the respective control for each condition. ( e ) The graph indicates the assembly sizes (average assembly area) for each condition as fold increase over their respective control conditions. ( d , e ) n =3–5 independent experiments, means±s.e.m. for all treatments, except for the knockdown (KD) conditions, where means±range of values (from two independent experiments) are shown. Data analyses are explained in the Supplementary Methods . The strongest increases in size are seen under treatments of low ionic strength, SPMAse, latrunculin A or cytochalasin D, all of which affect the membrane actin cytoskeleton. Full size image Although the overall area covered by protein assemblies was not strongly affected ( Fig. 5d ), several of the treatments indicated above had an effect on protein assembly size ( Fig. 5e ). The most evident effects were measured for the actin-depolymerizing drugs (latrunculin A and cytochalasin D), and for low ionic strength and SPMase treatments. Low ionic strength buffer and SPMAse incubation caused a loss of 71±7% and 85%±6% of membrane actin, respectively (compared with the sonication buffer incubation control, mean±s.e.m., n =3 independent immunostaining experiments; see also ref. 34 for the effects of SPMase on the actin cytoskeleton). These two conditions also caused an almost complete loss of spectrin, another important element of the membrane skeleton (after these treatments, immunostaining for spectrin gave signal intensities at or below the background level, n =2 independent experiments). Therefore, it appears that all treatments that increased the size of protein assemblies had either direct or indirect actin perturbation in common. Altogether, these observations suggest that the membrane-associated cytoskeleton is important for maintaining the protein assemblies apart from each other, or for limiting their size. However, the cytoskeletal elements are not essential for the persistence of the protein assemblies. These data also provide a potential explanation for the larger size of protein assemblies in membrane sheets, when compared with living membranes ( Fig. 3b ). Although there is an abundant actin staining on the membrane sheets ( Supplementary Fig. 3d , see also ref. 35 ), a partial loss of the filamentous actin network might trigger an increase in assembly size. The protein assembly pattern depends largely on cholesterol A much stronger effect on the membrane pattern was observed when we turned to the cholesterol depletion of membrane sheets. The entire assembly organization was eliminated by the removal of cholesterol via methyl-β-cyclodextrin (MBCD; Fig. 6a ). This effect was observed directly after 5–15 min incubations with MBCD (5–7.5 mM). The simplest interpretation of this phenomenon is that proteins diffused out of the assemblies, resulting in a much more homogeneous distribution. Small fluorescent puncta (below ~60 nm) were still occasionally visible, suggesting that some protein clusters survive this treatment. These are probably stabilized by cholesterol-independent mechanisms, such as specific protein–protein interactions. 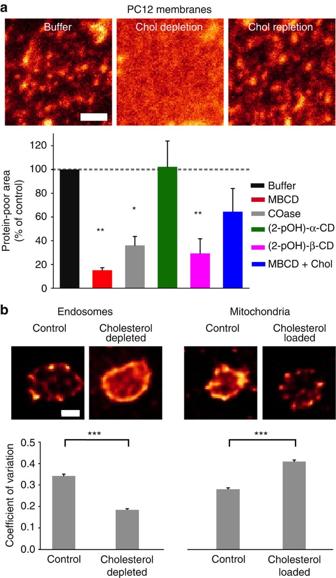Figure 6: Cholesterol controls the formation of protein assemblies. (a) The panels show STED images of PC12 membrane sheets treated with sonication buffer (left; 15 min at 37 °C), or subjected to cholesterol depletion with MBCD (middle; 5 mM, 5 min, followed by incubation in sonication buffer for 10 min at 37 °C). To replete cholesterol, after treatment with MBCD (5 mM, 5 min), cholesterol was loaded by applying MBCD-cholesterol (right; 5 mM, 10 min). Scale bar, 500 nm. To quantify the effects, we calculated the area occupied by assemblies as inFig. 5dbut here refer to the area poor in protein, as a an indication for the loss of assemblies. This fraction is predicted to be 0 on the complete dispersion of proteins from the assemblies. All values were expressed as % of control (buffer incubation alone). The bars show the following treatments: MBCD treatment as above, 0.2 units ml−1cholesterol oxidase (COase) for 15 min, 25 mM alpha- or beta-hydroxypropyl-CD for 5 min, cholesterol replenishment as above.n=3–7 independent experiments (*P<0.05; **P<0.01, 1-way analysis of variance, Dunnett’s multiple comparison test). The variance of the data was similar (0.34, 0.24, 0.44, 0.33, 0.37 and 0.74, for the six conditions, respectively). Note the loss of protein-free areas on cholesterol depletion, and their reformation (along with protein assemblies) on cholesterol repletion. (b) STED images of a normal (control) early endosome and of an early endosome treated with MBCD (left panels). STED images of a control mitochondrion and of a mitochondrion after loading with cholesterol (right panels). The images were processed by deconvolution for display purposes. Scale bar, 250 nm. The graph shows the quantification of the clustering of membrane proteins in endosomes and mitochondria, based on the coefficient of variation in fluorescence intensity along the line scans over the organelle membranes.n>110 organelles per condition, from multiple independent experiments (***P<0.001, two-sample Kolmogorov–Smirnov tests; this test was chosen since not all data sets passed a Jarque–Bera normality test). The variance of the data was similar (0.33, 0.54, 0.27 and 0.24, for the four data sets, respectively). SeeSupplementary Methodsfor the preparation and treatment of organelles. Figure 6: Cholesterol controls the formation of protein assemblies. ( a ) The panels show STED images of PC12 membrane sheets treated with sonication buffer (left; 15 min at 37 °C), or subjected to cholesterol depletion with MBCD (middle; 5 mM, 5 min, followed by incubation in sonication buffer for 10 min at 37 °C). To replete cholesterol, after treatment with MBCD (5 mM, 5 min), cholesterol was loaded by applying MBCD-cholesterol (right; 5 mM, 10 min). Scale bar, 500 nm. To quantify the effects, we calculated the area occupied by assemblies as in Fig. 5d but here refer to the area poor in protein, as a an indication for the loss of assemblies. This fraction is predicted to be 0 on the complete dispersion of proteins from the assemblies. All values were expressed as % of control (buffer incubation alone). The bars show the following treatments: MBCD treatment as above, 0.2 units ml −1 cholesterol oxidase (COase) for 15 min, 25 mM alpha- or beta-hydroxypropyl-CD for 5 min, cholesterol replenishment as above. n =3–7 independent experiments (* P <0.05; ** P <0.01, 1-way analysis of variance, Dunnett’s multiple comparison test). The variance of the data was similar (0.34, 0.24, 0.44, 0.33, 0.37 and 0.74, for the six conditions, respectively). Note the loss of protein-free areas on cholesterol depletion, and their reformation (along with protein assemblies) on cholesterol repletion. ( b ) STED images of a normal (control) early endosome and of an early endosome treated with MBCD (left panels). STED images of a control mitochondrion and of a mitochondrion after loading with cholesterol (right panels). The images were processed by deconvolution for display purposes. Scale bar, 250 nm. The graph shows the quantification of the clustering of membrane proteins in endosomes and mitochondria, based on the coefficient of variation in fluorescence intensity along the line scans over the organelle membranes. n >110 organelles per condition, from multiple independent experiments (*** P <0.001, two-sample Kolmogorov–Smirnov tests; this test was chosen since not all data sets passed a Jarque–Bera normality test). The variance of the data was similar (0.33, 0.54, 0.27 and 0.24, for the four data sets, respectively). See Supplementary Methods for the preparation and treatment of organelles. Full size image The effects of MBCD were reproduced by cholesterol oxidase and by a chemically different β-cyclodextrin, but not by a structurally related α-cyclodextrin [36] , which is unable to extract cholesterol ( Fig. 6a ). Importantly, cholesterol replenishment after MBCD treatment resulted in a major recovery of the membrane patterning ( Fig. 6a ; note the same phenotype in COS-7 cells, Supplementary Fig. 4 ), suggesting that the cholesterol influence is very strong compared with other factors (lipids and peripheral or cytoskeletal proteins) that might be lost during cholesterol depletion. We also verified the importance of cholesterol in other cellular membranes. We obtained organelles from AHA-treated PC12 cells, and manipulated their cholesterol level before fixation and click reaction. As in the plasma membrane, proteins were clustered in the membranes of early endosomes, and cholesterol depletion caused their dispersion ( Fig. 6b ). Mitochondrial membranes, which contain 40-fold lower levels of cholesterol than the plasma membrane [37] , had a more homogeneous protein distribution. Loading them with cholesterol-induced heterogeneities in protein distribution ( Fig. 6b ). This suggests that cholesterol has wide-ranging effects in membrane protein patterning, and that it is able to act even in membranes where it is not normally present at high levels. Nanoscale profiles of specific proteins in the assemblies Having thus determined the factors that maintain the organization of protein assemblies in the plasma membrane sheets, we proceeded to investigate the arrangement of individual proteins within the assemblies. We probed several integral and peripheral protein components of the membrane by immunostaining click-labelled membrane sheets (listed in Supplementary Table 1 ). The target proteins included transmembrane, acylated and peripheral membrane proteins, as well as cytoskeletal proteins from different functional protein classes, including those involved in neurotransmitter release (exocytosis), constitutive secretion, membrane recycling and cytoskeletal modifications ( Supplementary Table 1 ). All of the investigated proteins were present within the protein assemblies, both in PC12 and in COS-7 cells ( Fig. 7a and Supplementary Fig. 4b ). Most proteins were present only in some subsets of the assemblies, and within the assemblies they were further sub-segregated into nanoclusters. To determine the average location of the proteins within the assemblies, we performed line scans centred on the protein assemblies ( Fig. 7b ). The line scans revealed that many proteins had a preferential enrichment in particular areas: some were present mostly at the centres of protein assemblies; others preferred their edges, while some had no particular preference and were randomly distributed within the assemblies ( Fig. 7b ). Importantly, individual protein species had the same preference in PC12 or COS-7 cells ( Supplementary Fig. 4b ). 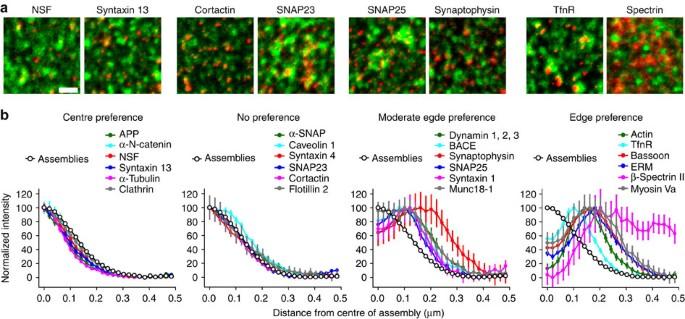Figure 7: Distributions of several proteins within the protein assemblies. (a) Selected proteins were fluorescently labelled through immunostaining (labelled red) on AHA-containing (labelled green) PC12 plasma membranes. The STED images indicate that all of these proteins co-localize with the assemblies to a good extent, but are enriched in different positions relative to assembly centres. Scale bar, 750 nm. (b) Analyses of the distributions of specifically labelled proteins, relative to the assembly centres. Protein distributions were categorized based on the widths of their profile: proteins having a tighter distribution (smaller full width at half maximum) than the general protein labelling were placed in the ‘Centre preference’ category, while those that had similar distributions to the protein assemblies were described as ‘No preference’ (no preferred distribution within the assemblies). Protein distributions whose peak was away from the centre of the protein assemblies were categorized according to the ratio between their intensity at the centre of the protein assembly and their peak intensity. Those where the central point represented more than 60% of the peak value were described as having a ‘Moderate edge preference’, while those where the central point was below this value were described as having an ‘Edge preference’. The graphs indicate averaged normalized line scans, from 300–900 protein assemblies (mean±s.e.m.). The line scan profile for the assemblies (average for all stainings in each category) is shown in black (hollow circles), as a reference. SeeSupplementary Fig. 3bfor stainings on COS-7 membranes, andSupplementary Fig. 5for control stainings with different types of probes, and under different sample preparation conditions. Figure 7: Distributions of several proteins within the protein assemblies. ( a ) Selected proteins were fluorescently labelled through immunostaining (labelled red) on AHA-containing (labelled green) PC12 plasma membranes. The STED images indicate that all of these proteins co-localize with the assemblies to a good extent, but are enriched in different positions relative to assembly centres. Scale bar, 750 nm. ( b ) Analyses of the distributions of specifically labelled proteins, relative to the assembly centres. Protein distributions were categorized based on the widths of their profile: proteins having a tighter distribution (smaller full width at half maximum) than the general protein labelling were placed in the ‘Centre preference’ category, while those that had similar distributions to the protein assemblies were described as ‘No preference’ (no preferred distribution within the assemblies). Protein distributions whose peak was away from the centre of the protein assemblies were categorized according to the ratio between their intensity at the centre of the protein assembly and their peak intensity. Those where the central point represented more than 60% of the peak value were described as having a ‘Moderate edge preference’, while those where the central point was below this value were described as having an ‘Edge preference’. The graphs indicate averaged normalized line scans, from 300–900 protein assemblies (mean±s.e.m.). The line scan profile for the assemblies (average for all stainings in each category) is shown in black (hollow circles), as a reference. See Supplementary Fig. 3b for stainings on COS-7 membranes, and Supplementary Fig. 5 for control stainings with different types of probes, and under different sample preparation conditions. Full size image Since antibody-induced clustering is a serious issue in protein imaging [38] , we verified the protein distributions on membrane sheets with smaller, monovalent probes, such as fluorophore-coupled Fab fragments or single-chain variable domains for syntaxin 1 and tubulin, respectively ( Supplementary Fig. 5a ), or an RNA aptamer for the transferrin receptor ( Supplementary Fig. 5b ). Finally, transferrin receptor, an edge-preferring protein, was shown to remain at the edges of the enlarged protein assemblies that form after treatment of membrane sheets with low ionic strength buffer ( Supplementary Fig. 6a ). We conclude that different proteins prefer individual areas in protein assemblies. This pattern is robust, as it is maintained in different cell types, and even after treatments that modify the assembly size. Functional partners favour similar regions of the assemblies Distribution within the assemblies appeared to be strongly influenced by characteristics specific to each protein. For example, although palmitoylated proteins generally occupied assembly centres ( Fig. 4b ), one member of this class, SNAP25, had a moderate preference for assembly edges ( Fig. 7 ). It is possible that the interaction partner syntaxin 1, which is located at the periphery, pull SNAP25 nanodomains to the periphery through specific protein–protein interactions. In fact, this view is further supported by the observation that a truncated version of SNAP25, lacking the SNARE domains required for syntaxin 1 interaction and expressed in COS-7 cells where neuronal interactions partners are missing, lost the preference for assembly edges ( Supplementary Fig. 6b ). This suggests that interactions specific to the SNARE domains, and not just palmitoylation, contribute to the distribution of SNAP25. An inspection of the different groups of proteins in Fig. 7b suggests that several functional partners are co-localized. For example, actin preferred a region at a distance of ~150 nm from the centres ( Fig. 7b ). Here, it was joined by functional partners like myosin and actin-plasma membrane linking ERM (ezrin–radixin–moesin) proteins [39] , which participate in the organization of the so-called ‘membrane skeleton [20] ’. The ring-like distribution of actin ( Supplementary Fig. 3d ), seemingly forming a barrier (or border) at the edges of the assemblies, is in line with the effects of actin disruption ( Fig. 5 ). Spectrin also avoided the assembly centres. Unlike actin, which was present on the assembly borders, spectrin occupied not only the assembly edges, but also penetrated into the space between them. This suggests that spectrin, together with actin, may participate in spacing the protein assemblies in the plasma membrane, as suggested for the organization of axonal domains [40] . A cohort of proteins (SNAP25, syntaxin 1, bassoon, synaptophysin, their co-factor lipid phophatidyl-inositol 4,5-bisphosphate) involved in the fusion of neurotransmitter-containing vesicles to the plasma membrane (Ca 2+ -regulated exocytosis) localized to assembly edges ( Figs 4d and 7 ). In contrast, SNAP23 and syntaxin 4, which are involved in the fusion of vesicles from the constitutive secretion pathway, displayed more random distributions, despite their remarkable structural similarity to SNAP25 and syntaxin 1. The endosomal proteins amyloid precursor protein and syntaxin 13 both preferred assembly centres. Further examples of proteins that seem to localize to similar areas are the functionally related sorting proteins NSF and α-SNAP, which are involved in the disassembly of SNARE complexes following membrane fusion. These observations suggest that the nanoscale organization of specific proteins is superimposed on the general mesoscale protein assembly pattern. We provide here a comprehensive survey of general protein distribution in living cells and plasma membrane sheets from two different cell lines. We demonstrate that long-lived (lasting for minutes to tens of minutes), relatively stable protein assemblies exist in the plasma membrane of living cells ( Figs 1 and 2 ). Although a substantial population of proteins are highly mobile, many proteins were found in assemblies in which protein diffusion is limited ( Fig. 1d , FRAP measurements and Fig. 1e,g , STED-FCS). Using membrane sheets to determine the organizational principles of the assemblies, we found that they enrich a variety of proteins ( Fig. 4 ), which occupy different positions ( Fig. 7 ). The assemblies are dependent on cholesterol ( Fig. 6 ), and are bordered by both actin and spectrin ( Fig. 7 and Supplementary Fig. 3d ). Elimination of these cytoskeletal elements results in an increase the assembly size ( Fig. 5 ). Besides many previous studies and models [12] , [15] , [21] , [41] , [42] , these results are also largely in agreement with a systematic high-resolution imaging study of green fluorescent protein-coupled membrane proteins in living yeast cells [43] , which also found that modifications of sterol composition affected the distribution of all proteins, while actin disruption had less dramatic effects. The localization within the assemblies, as well as the extent of enrichment in the assemblies, was quite variable for different anchors ( Fig. 4b ) and for different protein species ( Fig. 7 and Supplementary Table 1 ). This implies that despite the general enrichment of almost all of the tested proteins within assemblies, specific protein–protein and protein–lipid interactions are important for further segregation processes, which define the functional composition of the assemblies, as well as that of protein-poor regions. Our results fit with and complement two major lines of investigation of membrane composition. On one hand, several studies of osmium-stained membrane sheets showed a patchwork of light and dark areas, with several specific proteins enriched in the latter [14] , [15] , [16] , [44] , [45] . On the other hand, nanoscale clusters have been reported for many proteins over the years, using techniques ranging from immunogold labelling to live-cell super-resolution microscopy [1] , [14] , [18] , [46] , [47] . We suggest that protein assemblies are the structure behind the previously observed dark patches, and that nanoscale domains of different proteins form within the protein assemblies. However, many of the previous observations of patchwork protein patterns were made using isolated membrane sheets, giving rise to concerns regarding artefactual protein aggregation. Increased aggregation has indeed been demonstrated [35] , albeit on membranes incubated for tens of minutes with millimolar concentrations of calcium, which probably induced much of the aggregation [35] , [48] . We show here that protein-rich assemblies do exist in living cells under physiological conditions ( Fig. 1 ). Nevertheless, the assemblies can be more evident in membrane sheets, likely due to the loss of cytoskeletal elements during long incubations (which leads to increases in protein assembly size as shown by actin disrupting drugs Fig. 5e ). An argument against the formation of protein patterns in living cells has been the claim that protein distributions in rapidly frozen membranes are homogeneous, as in the classical electron microscopy studies of Heuser, Reese and collaborators [49] , [50] . This latter argument may not be fully correct. We analysed the distribution of intramembrane particles (proteins) in several images from these studies, and found them to be distributed in a non-random fashion ( Supplementary Fig. 7a ). To allow for a visual comparison of the electron microscopy data with fluorescence microscopy experiments, we replaced the protein positions with fluorescent labels in silico ( Supplementary Fig. 7b ). A patchy pattern is evident, resembling distribution of proteins shown in Figs 1b , 3a . For a quantitative comparison, we analysed the in silico generated fluorescence images as in Fig. 7 (see Supplementary Fig. 7c ). We compared the results with a similar analysis of live STED images of COS-7 cells, which should be closer to the rapidly frozen situation than fixed cells. The resulting enrichment profiles were similar, despite the widely different techniques used in these experiments ( Supplementary Fig. 7c ). Importantly, the fact that similar protein distributions are found for fibroblast membranes (our work) and in the membrane of frog presynaptic boutons (Heuser, Reese and collaborators) points to the general applicability of the protein assembly pattern. Among all of the factors tested, cholesterol seemed to be the main stabilizer of protein assemblies, as its removal dissipated the proteins, in a reversible fashion ( Fig. 6 ). This general effect of cholesterol is not fully surprising, since major changes in membrane properties have been previously shown in model membranes and in cells in response to cholesterol depletion [18] , [42] , [51] , [52] , [53] . The exact mechanism remains speculative. At least two main scenarios can be envisioned, which could take place simultaneously. First, a subset of membrane proteins may be enriched in cholesterol-induced lipid domains, as suggested by the ‘lipid raft’ hypothesis [54] . In agreement with this hypothesis, our results show a preferential enrichment of raft-preferring proteins in the centres of the protein assemblies (palmitoylated and GPI-anchored proteins; Fig. 4b and Supplementary Fig. 2 ). It is conceivable that during density gradient centrifugation, after Triton solubilization, the centres of such assemblies may remain non-solubilized, and may therefore float up. Second, a subset of transmembrane proteins might be driven into protein assemblies by unfavourable lipid solvation of their transmembrane domains in presence of high cholesterol concentrations. This is in line with studies on membrane peptides in artificial systems, which showed that the physiological levels of cholesterol significantly increase membrane thickness and at the same time stiffen lipid acyl chains, thus causing the segregation of proteins into protein-rich domains where protein–protein contacts are increased [55] , [56] , [57] . Also, the lipid shell concept suggests a similar effect from the perspective of high density of proteins inducing local lipid disturbances [58] . In addition to these rather unspecific effects of cholesterol, more direct cholesterol–protein interactions might also contribute to the assembly organization. Many scaffolding proteins have been found to contain a cholesterol-recognition amino acid consensus motif that allows specific binding to cholesterol, which in turn modulates the protein function and distribution [59] , [60] . Finally, we would also like to point out that in our work on cholesterol depletion experiments have been performed in isolated membrane sheets or endosomes, since this procedure is highly toxic to living cells, and since other side effects and compensatory mechanisms would be triggered in living cells, which would complicate any interpretation. We therefore cannot neglect the possibility that the potential loss of other components in the membrane sheets might render them more open to the action of cholesterol depletion, in comparison with living cells. In addition to cholesterol, the membrane cytoskeleton is also involved in the organization of protein assemblies, by bordering them ( Figs 5c,e and 7b and Supplementary Fig. 3d ). Our observations are therefore in agreement with the ‘actin picket fence’ model and the ‘hop-diffusion’ behaviour proposed for both proteins and lipids in the membrane [20] , [21] . According to this model, protein diffusion is confined within membrane compartments bordered by a ‘picket actin fence’, but occasionally the proteins may ‘hop’ from one compartment to another [61] . In addition to this model, the confinement of the proteins in the assemblies may lead to intensified protein–protein interactions and to a lower diffusion in the high-density areas, which will contribute to the hop-diffusion behaviour (see also ref. 62 ). We suggest that protein assemblies might have a facilitative role in the establishment of functional, more specific interactions. A main advantage of enriching proteins in the assemblies could be to provide spatiotemporal regulation to signalling events, to dynamic functions such as exo-/endocytosis, or to enzymatic reactions. Interestingly, a recent simulation study suggested that confinement of proteins in membrane domains facilitates reaction bursts instead of low yield constant reactions, which would take place in a uniform membrane [63] . In addition to this general effect on membrane reactions, protein sub-compartmentalization in assemblies may support specific functions. As suggested in Fig. 7 , several proteins involved in the regulated exocytosis of synaptic-like microvesicles or neurotransmitter filled dense-core vesicles [64] co-localize at the edges of the assemblies, probably enabling the rapid and efficient fusion of these vesicles in the less crowded areas between the assemblies. In contrast, SNAP23 and syntaxin 4, which are involved in the slower constitutive secretion, are not preferentially located to such sites. Localization can also be easily understood in functional terms for synaptophysin, a component of synaptic vesicles and microvesicles [64] , that is also enriched at the edges of assemblies. This location is ideal for it to be retrieved from the plasma membrane by endocytosis, without much interference from many other membrane proteins. Regarding this view, it might be contradictory that proteins of the endocytotic machinery, such as clathrin and caveolin appear not to show strong edge preference. However, it is probable that membrane-attached clathrin and caveolin are found mostly in coated pits that are uniformly covered with these molecules, in a way creating their own specialized assemblies, with a defined function (endocytosis). Finally, protein assemblies may also serve to remove the reactivity of certain proteins, keeping them in a less mobile, and perhaps less reactive state. In fact, for syntaxin 1 it has been shown that clustered molecules are less reactive than those diffusing freely [65] . Therefore it is tempting to speculate that protein assemblies reduce the effective concentration of at least some membrane proteins. We conclude that the enrichment of plasma membrane proteins in multi-protein assemblies is a fundamental principle that creates a mesoscale organization with important functional implications, at various levels. Cells and membrane sheets Coverslips were sequentially washed with 1 M NaOH, 1 M HCl and 100% ethanol. PC12 and COS-7 cell lines were kindly provided by Reinhard Jahn (Max Planck Institute of Biophysical Chemistry, Göttingen, Germany). PC12 cells were cultured on poly-L-lysine (PLL)-coated coverslips as described before [33] . For AHA labelling, cells were incubated for 3 days in medium (Dulbecco’s Modified Eagle’s Medium (DMEM), high glucose, no glutamine, no methionine, no cysteine; from Gibco) complemented with 4 mM glutamine, 10% dialysed horse serum (Biochrom), 5% dialyzed fetal calf serum (PAA), 0.6% penicillin-streptomycin, 50 μM L -azidohomoalanine (Click-iT AHA from Invitrogen) and 400 μM cysteine. Membrane sheets were generated by exposing cells to a brief ultrasound pulse using a Sonoplus sonifier (Bandelin) at 65–75% of the full power, in ice-cold sonication buffer made of 120 mM potassium glutamate, 20 mM potassium acetate, 10 mM EGTA, 4 mM MgCl 2 , 2 mM ATP, 0.5 mM DTT, 20 mM HEPES-KOH, pH 7.2 (ref. 66 ). The membrane sheets were then washed with K-Glu buffer (120 mM potassium glutamate, 20 mM potassium acetate, 10 mM EGTA, 4 mM MgCl 2 , 20 mM HEPES-KOH, pH 7.2). Membrane protein organization in membrane sheets is expected to be similar to intact cells, as documented by unaltered membrane protein diffusion [1] and by similar membrane protein patterning [11] . Membrane sheet treatments were performed with the concentrations of reagents and incubation times indicated in the figure legends. All incubations were done at 37 °C, unless otherwise stated. For each experiment, we prepared control samples that were incubated with the sonication buffer alone (or with the solvent used for drug applications; typically dimethyl sulfoxide) for the same time intervals. COS-7 cells were cultured as described before [67] and were grown for 3 days with AHA, as above (with 10% dialyzed fetal calf serum and no horse serum). All further experiments with COS-7 cells were performed as for PC12 cells. After sonication, PC12 and COS-7 membrane sheets were either fixed with 4% PFA+0.2% glutaraldehyde at room temperature (RT) for 45 min ( Figs 2 and 4a–c , and Supplementary Figs 2 and 6b ), or with 4% PFA for 10 min on ice and another 30 min at RT ( Figs 3a , 4d and 5 , 6 , 7 , and Supplementary Figs 3, 4, 5a and 6a ), unless otherwise noted in the figure legends. They were then quenched with 100 mM NH 4 Cl in PBS for 25 min at RT. Unless otherwise indicated, click reactions on membranes were performed after fixation and quenching, as described below. See below for various treatments of membrane sheets ( Figs 5 and 6 ). Ionic alterations After sonication, membrane sheets were incubated for 20 min in high-salt buffer (sonication buffer containing 500 mM KCl), low ionic strength buffer (320 mM sucrose, 5 mM HEPES-KOH, pH 7.2) or high-calcium buffer (sonication buffer containing 1 mM Ca 2+ ). Alternatively, cells were incubated with 1 μM ionomycin (Sigma) for 5 min in HEPES-buffered DMEM (Gibco), in the presence of 5 mM CaCl 2 , with or without 10 mM EGTA. Membrane sheets were obtained from the treated cells after three brief washes with HEPES-buffered DMEM. Cytoskeleton disruptions Before sonication, cells prelabelled with AHA for 3 days were incubated for 1 h in the AHA-incubation medium described above, containing 10 μM nocodazole (Sigma), 10 μM colchicine (Sigma), 1 μM latrunculin A (Calbiochem), 10 μM cytochalasin D (Sigma) or 0.1% dimethyl sulfoxide (as solvent control). They were then washed and subjected to sonication, followed by fixation with 4% PFA. Lipid perturbations For sphingomyelin removal, membranes were incubated with 20 units ml −1 SPMase (Sigma) for 15 min at 37 °C, washed and fixed. The following phospholipases (PL; from Sigma) were similarly applied in the following final concentrations: 2 units ml −1 of PLA2 from bovine pancreas, 2 units ml −1 of PLC from Clostridium perfringens , 1 unit ml −1 of phosphatidylinositol-specific (PI-specific) PL-C from Bacillus cereus and 2 units ml −1 of PLD from Streptomyces sp. For cholesterol depletion, membranes were incubated for 5 min with 5 mM MBCD (Sigma), dissolved in sonication buffer at 37 °C. This step was followed by three fast washes with buffer, and by either a 10-min incubation in sonication buffer at 37 °C or a 10-min incubation in sonication buffer containing cholesterol complexed with 5 mM MBCD at 1:10 molar ratio (for membrane repletion with cholesterol), as described previously [68] . Alternatively, membranes were incubated with 0.2 units ml −1 cholesterol oxidase (Sigma) for 15 min, or with 25 mM (2-Hydroxypropyl)-α-CD (Sigma-Aldrich) or (2-Hydroxypropyl)-β-CD (Sigma) for 5 min at 37 °C; this was followed by three washes and a 10-min incubation in sonication buffer (to keep the total incubation time constant across different conditions). For each condition, controls were prepared by incubating the membrane sheets in sonication buffer alone at 37 °C for the same duration of the respective treatment. Click reactions In copper-free click reactions, AHA (Invitrogen) was coupled to 40 μM DIBAC-KK114. The reaction was allowed to proceed for 1 h at 37 °C, in PBS containing 1.5% fetal calf serum. Cells were washed several times with PBS containing 3% fetal calf serum, both before and after the reactions. The labelling was performed in plastic cell culture dishes, and the cells were then suspended by application of cold PBS containing 10 mM EDTA, and were plated on PLL-coated coverslips. The cells were allowed to adhere in normal DMEM with 10% fetal calf serum for 1 h, before live imaging at 37 °C in DMEM without phenol red. In copper-catalysed click reactions, AHA was coupled to 2 μM Atto647N-alkyne (Atto-tec), using the Click-it Cell Reaction Buffer Kit according to the manufacturer’s protocol (Invitrogen). In two-colour STED experiments AHA was coupled to 5 μM Chromeo494-alkyne (Active Motif), following the same protocol. To block or remove unspecific binding to the membranes, we washed fixed preparations for 15 min with PBS (137 mM NaCl, 2.7 mM KCl, 10 mM Na 2 HPO 4 , 2 mM KH 2 PO 4 , pH 7.4) containing 5% bovine serum albumin (BSA) and 5% peptone, and briefly with PBS containing 3% BSA, both before and after the reaction. In cases where L-HPG (Invitrogen) was used as an alternative methionine analogue, azide-functionalized versions of the same fluorescent dyes were used. Click labelling of post-translational protein modifications was performed similarly. Click labelling of post-translational protein modifications During the 3-day AHA or HPG incubation for protein labelling, PC12 cells were additionally incubated with one of the following metabolic labelling reagents purchased from Invitrogen: 200 μM palmitic acid azide for 24 h, 50 μM myristic acid azide for 24 h, 50 μM geranylgeranyl alcohol azide for 24 h, 50 μM farnesyl alcohol azide for 48 h, 50 μM tetraacetylfucose alkyne (fucose-alkyne) for 72 h, 50 μM tetraacetylated N-azidoacetyl- D -mannosamine (ManNAz) for 72 h, 50 μM tetraacetylated N-azidoacetylglucosamine (GlcNAz) for 72 h, and 50 μM tetraacetylated N-azidoacetylgalactosamine (GalNAz) for 72 h (if not present all the time, the reagents were added towards the end of the 3-day incubation). Two click reactions were performed sequentially on membrane sheets obtained from these cells (separated by thorough washes), the first to label the proteins with Chromeo494, and the second to label the protein modifiers with Atto647N. Microscopy Leica TCS SP5 STED microscope (Leica Microsystems), equipped with a × 100 1.4 NA PL APO CS oil objective (Leica) was used for the FRAP experiment in Fig. 1d and all the subsequent figures with fixed samples. The excitation of Atto647N, KK114 or Star635 was performed using a pulsed diode laser (Leica Microsystems) at 635 nm. In STED mode, depletion was achieved by means of a Spectra-Physics Mai Tai tunable laser (pulsed at 80 MHz; Titanium Sapphire, Newport Spectra-Physics) at 750 nm,. For two-colour STED, Chromeo494 was excited with a pulsed diode laser at 535 nm and the same depletion laser was used for STED effect. For confocal images, the following excitation lines were used: an Argon laser at a wavelength of 488 nm for green fluorescent protein and 514 nm for yellow fluorescent protein, and Helium–Neon lasers at 543 nm for rhodamine and 633 nm for KK114 or Atto647N. Signal detection was performed using photomultiplier tubes in confocal mode and an avalanche photodiode in STED mode. Laser intensities were adjusted to obtain the best signal-to-noise ratio for each experiment. The images are displayed with individual scaling, except for Fig. 1d , and Supplementary Figs 1a and 3a,b . The STED resolution was ~40–50 nm when measuring Atto647N (red channel). Measurements with Chromeo494 (green channel) were performed at a resolution of ~80 nm. For living cells, imaging was performed at 37 °C. Single- and two-colour live-cell measurements with Chol-PEG-490LS and DIBAC-KK114 ( Fig. 1b,c,e–g ) were performed on the scanning STED-FCS setup described below. Briefly, Atto490LS and KK114 were excited with 490 nm and 635 nm pulsed laser diodes, respectively. The stimulated emission of both dyes was induced at 780 nm with a Ti:Sa laser with an average power of 100 mW in the back aperture of the objective. We found that the optimal imaging conditions to detect the protein assemblies were to use a resolution of 70 nm for red channel (proteins), which corresponds to 90 nm for the green channel (Chol-PEG-490LS), and short pixel dwell times between 10 and 20 μs. Except Fig. 1c , two-colour STED images in the figures are processed by median filtering for display. Scanning STED-FCS measurements and analysis The optical setup for the STED-FCS measurements and the data analysis was described before [30] , [69] . Here, we applied a scanning FCS scheme similar to the one described in Digman and Gratton, 2009 (ref. 29 ). Circular trajectories with a diameter of 1.2 μm were scanned on the basal (bottom) plasma membrane at 37 °C with a frequency of 4 kHz. The STED power applied in the back aperture of the objective was 40 mW (780 nm), resulting in an observation spot with a diameter of 90 nm (FWHM). The excitation power at 635 nm was 10 μW. The scanning trajectories were subdivided into 50 pixels and for each pixel a standard FCS analysis was performed using self-written Matlab routines. The temporal correlation functions were fitted according to the standard two-dimensional diffusion model. This analysis gives the average density and the average diffusion constant of the fluorescently labelled proteins simultaneously, for each pixel on the scanning trajectory. We used the Pearson correlation coefficient analysis to test whether protein density correlated with the diffusion constant. The values of the Pearson correlation coefficient can range from 01 to −1, that is, from strong positive correlation (diffusion is faster in protein assemblies) to strong negative correlation (diffusion is slower inside the protein assemblies). Note that our FCS analysis omits all molecules that are very slow ( D <0.01) or non-moving. FRAP After a 3-day incorporation of AHA, COS-7 cells were labelled with DIBAC-KK114 by live copper-free click reactions (as detailed above), and were imaged in confocal mode at 37 °C, using the Leica TCS SP5 STED setup described above, with the Leica LAS FRAP Wizard (bleach point mode). After acquisition of three frames before bleaching (at 3.093 s per frame), bleaching was performed by applying the 633 and 635 nm lasers at full power for 1 s. This procedure results in bleaching a circular area, whose size was estimated as detailed below. Bleaching was followed by the acquisition of at least 30 post-bleaching frames, to measure recovery. The recovery curve was corrected for potential photobleaching during image acquisition, by using reference spots outside of the bleach area. To determine the diffusion coefficient, the corrected recovery curve was fit to a double exponential curve. Diffusion coefficients were calculated according to D = r 2 /4* t 1/2 where r is 1/ e 2 radius of the bleached area, and t 1/2 is the half-time of recovery [70] . To find the r for the circular bleached area, horizontal and vertical line scans were performed on the bleached position. The resulting averaged line scan was fit to a Gaussian curve to calculate the value of r , which was equal to 1.8 μm. Cell–cell fusion Two sets of COS-7 cells were grown with AHA or HPG for 60 h. They were then starved for methionine for 15 min, were suspended by application of cold PBS containing 10 mM EDTA and were plated together on PLL-coated coverslips and allowed to adhere overnight in normal COS-7 medium. To induce fusion, an inactivated Sendai virus extract was used (Sendai virus envelope, HVJ-E, supplied by Cosmo Bio, Tokyo, Japan, as HVJ Envelope Cell Fusion Kit GenomONE-CF Ex). Cells were allowed to adsorb HVJ-E for 5 min on ice. After washing with the provided fusion buffer, cells were left in fusion buffer at 37 °C for 16 min, to trigger fusion. Afterwards, the cells were kept in normal COS-7 medium at 37 °C for 5 or 60 min. All measured fluorescence intensities were corrected for fluorescence bleed-through and non-specific fluorophore background. As negative fusion controls, we used cells incubated under the same conditions, but in the absence of HVJ-E. No spontaneous exchange of labelled proteins was observed in this case. Intermixing of colours in the absence of HVJ-E was indistinguishable from fluorescence bleed-through and/or non-specific background. Transfer of lipid probes to the plasma membrane of living cells Stock solutions of 50 μM Chol-PEG-490LS were prepared in pure water containing 1% ethanol. Cells were then incubated with 200 μl of a 1:200 dilution of the stock in cell medium, for 3 min at RT. After incubation, the cells were washed with the medium. See Supplementary Methods for the preparation of PEGylated cholesterol probes. Incorporation of fluorescent lipids into membrane sheets In order to check the integrity of the membrane sheets after the click reaction, we labelled the membranes with 1 μg ml −1 octadecyl rhodamine B chloride (R18, Invitrogen) for 10 min; we then performed three washes with PBS (10 min each), and embedded the membrane sheets in Mowiol. R18 imaging was performed in confocal microscopy. Alternatively, more specific lipid analogues were used. A stock solution of 50 μM of Chol-PEG-KK114 was prepared in pure water containing 1% ethanol. A 100-μM stock solution of Atto647N-PE ( N -(Atto647N)-1,2-dipalmitoyl- sn -glycero-3-phosphoethanolamine with head group labelling) was prepared in 100 μM fat-free BSA water solution [69] . For imaging specific lipids, membranes were incubated (after click reactions) with Chol-PEG-KK114 or Atto647N-PE, diluted 1:100–200 from the stocks mentioned above, for 30 min at RT. The cells were then washed with PBS, fixed and embedded in Mowiol. Samples were imaged directly after preparation. Immunostaining of the membrane sheets After the click reaction, immunostainings were performed in PBS containing 1.5–3% BSA with primary antibodies for 1 h at RT, followed by washing and incubation with secondary antibodies for 1 h. The antibodies used are listed in Supplementary Methods . Data analysis All analyses were performed with the help of Matlab software (The Mathworks Inc.), using self-written routines. The routines are described, for each figure, in Supplementary Methods . How to cite this article: Saka, S. K. et al . Multi-protein assemblies underlie the mesoscale organization of the plasma membrane. Nat. Commun. 5:4509 doi: 10.1038/ncomms5509 (2014).